Paramagnetic relaxation enhancement NMR as a tool to probe guest binding and exchange in metallohosts Paramagnetic metallohost systems can bind guest molecules and find application as biomimetic catalysts. Due to the presence of the paramagnetic metal center, rigorous characterization of these systems by NMR spectroscopy can be very difficult. We report here that metallohost-guest systems can be studied by using the paramagnetic relaxation enhancement (PRE) effect. Manganese(III) porphyrin cage compounds are shown through their PRE to thread and bind viologen guests, including a polymeric one. The binding constants and dethreading activation parameters are lower than those of the metal-free porphyrin cage compounds, which is proposed to be a result of charge repulsion of the trivalent metal center and dicationic viologen guest. The threading rate of the manganese(III) porphyrin cage onto the polymer is more than 10 times faster than that of the non-metallated one, which is ascribed to initial binding of the cage to the polymer chain prior to threading, and to an entron effect. NMR spectroscopy is a powerful tool in supramolecular chemistry, not only for characterizing host-guest systems and performing binding studies, but also for investigating the kinetics of host–guest exchange at equilibrium [1] , [2] , [3] , [4] , [5] . Diamagnetic systems are the simplest to study since they display sharp lines, allowing for a multitude of 1D and multidimensional techniques to be applied. Paramagnetic systems pose complications for studying host–guest interactions since chemical shift and nuclear relaxation can be greatly influenced by the presence of unpaired electrons. However, even these challenging properties can provide opportunities for answering chemical questions and be utilized to gain insight into exchange and binding processes. Here, we show that metallohost–guest binding and exchange in a paramagnetic manganese(III) porphyrin macrocycle can be studied by NMR spectroscopy by exploiting the paramagnetic properties of the metal center, i.e., by using the paramagnetic relaxation enhancement (PRE) effect. So far, PRE has been utilized by various NMR methods studying paramagnetic systems such as characterization by means of hyperfine shifts [6] , [7] , [8] , measurement of protein–ligand kinetics via dissolution dynamic nuclear hyperpolarization (DNP) [9] , studying Xe host-guest complexes via paramagnetic hyper-CEST [10] , [11] , paramagnetic GEST (host–guest variant of CEST) combining MRI and NMR [12] , and diffusion NMR (DOSY) [13] , [14] . Furthermore, a toolbox using standard NMR techniques has been reported in the characterization of paramagnetic compounds [15] . In biochemistry, PRE has mainly been applied for the study of enzyme mechanisms [16] , [17] , [18] , protein structure characterization [19] , [20] , [21] , [22] , drug discovery [23] , [24] , [25] , [26] , [27] , and protein dynamics and exchange reactions [28] , [29] , [30] , [31] , [32] , [33] . To the best of our knowledge PRE NMR has not been used to study association and dissociation phenomena in organic and supramolecular chemistry. The studies presented here are part of an overarching project aimed at the development of manganese(III) porphyrin macrocyclic catalysts that can thread onto a polybutadiene chain, and while moving along it, convert the polymer double bonds into epoxides [34] , [35] . In previous work, we studied the mechanism of exchange of small N , N ′-dialkyl-4,4′-bipyridinium (viologen) guests as well as polymers containing a viologen moiety in diamagnetic (metal-free or Zn) porphyrin macrocycles through UV–Vis, fluorescence, and EXSY NMR spectroscopy [36] . Unfortunately, spectroscopic studies on the actual catalytic system, i.e., the Mn(III)-porphyrin macrocycle, have not been possible, and as a result the effect of the Mn center in the porphyrin on exchange and binding has not yet been determined. This is due to the lack of fluorescent properties of Mn porphyrins, inconclusive UV–Vis behavior, and short T 2 s, which cause unmanageably broad peaks in the 1 H NMR spectra, making EXSY studies impossible to perform. Hence, we decided to study the dynamics of the actual host–guest system by measuring the PRE on an excess of free viologen guests, including both low molecular weight and polymeric ones ( V1 , V2 and VP , see Fig. 1 ), which are exchanging at equilibrium with the bound host Mn(III)-porphyrin macrocycle Mn1 . In this work, we provide a clear-cut NMR spectroscopic method to study exchange in these paramagnetic host–guest systems and to determine the threading and binding parameters involved. We show that manganese(III) porphyrin cage compound Mn1 can thread and bind viologen guests, including a polymeric one. The binding constants and de-threading activation parameters unexpectedly are lower than those of the metal-free porphyrin cage compound H 2 1 . Furthermore, the threading rate of Mn1 onto the polymer is much faster than that of H 2 1 , which is ascribed to initial binding of the cage to the polymer chain prior to threading, and to an entron effect. Fig. 1: Molecular structures of the studied compounds. Mn(III)-porphyrin cage compound Mn1 (porphyrin center atom(s) indicated in blue), bis-(methyl cyclohexyl) viologen V1 , methyl viologen V2 , polymer-substituted viologen VP , and the rotaxane of a blocked viologen guest (blue) with Mn1 ( MnRot ). Full size image In the presence of a paramagnetic center, an increase in the longitudinal ( R 1,obs (s −1 )) and transverse ( R 2,obs (s −1 )) relaxation rate of a given nucleus can be observed. This observed relaxation rate is defined as the sum of the diamagnetic ( R 0 ) and paramagnetic ( R p ) relaxation rates (Eq. 1 ). R 1,obs and R 2,obs can be determined by measuring the T 1 (s) and T 2 (s) values of a specific signal in a sample containing both the paramagnetic host and diamagnetic guest compound in solution. The terms R 1,0 and R 2,0 can be obtained by measuring the T 1 and T 2 values of this signal in a sample containing only the diamagnetic guest compound in solution. Exchange parameters can be calculated from R p , which, however, is dependent on the regime of exchange. R_obs=R_0+R_p
 (1) There are three regimes of exchange (fast, intermediate, and slow) with respect to nuclear relaxation that provide information about the interaction of a guest with a paramagnetic center. Here, we take advantage of PRE in two ways: (1) fast exchange of solvent inside an empty host to determine the association constant of viologen guest binding, and (2) slow, reversible dissociation of viologen guests to determine dissociation rate constants. Measuring the binding strength of paramagnetic host-guest systems The 1 H NMR spectrum of the diamagnetic metal-free porphyrin macrocycle H 2 1 gives well-defined and isolated sets of signals (Fig. 2 , top). However, when a Mn(III)-Cl center is inserted into the porphyrin ( Mn1 ), all host signals broaden due Fig. 2: Influence of the presence of a paramagnetic Mn center on the 1 H NMR spectrum of a host compound. Top: 1 H NMR spectrum of metal-free porphyrin cage compound H 2 1 (500 MHz, chloroform- d : acetonitrile- d 3 , 1:1 (v/v), 25 °C), bottom: 1 H NMR spectrum of Mn1 (500 MHz, chloroform- d : acetonitrile- d 3 , 1:1 (v/v), 25 °C) (metal center and counter ion in blue). Full size image to the paramagnetic effect of the metal center on the cage compound (Fig. 2 , bottom). The sharpest of the signals, near 7.0 ppm, correspond to the phenyl groups at the bottom of the cage, which are the farthest away from the Mn center and thus experience the least dipolar relaxation enhancement due to the r −6 distance component. In order to accurately calculate the exchange parameters of the host–guest systems, the population of bound host should be determined for each measured system, which can be calculated through the respective binding constants. Due to the difficulty of measuring binding through routinely-used spectroscopic techniques [36] , [37] , [38] , [39] , [40] , we resorted to biochemical NMR spectroscopy for inspiration, as our hosts mimic to some extent properties of metalloproteins and metalloenzymes. Claridge et al. have taken advantage of the change in R 1,obs of the bulk solvent water when it has access to a paramagnetic metal center buried inside a protein to determine the binding constant of a second, more competitive ligand to this metal center [41] . As soon as the competitive ligand binds to the metal center completely, the water will only be affected by the weaker outer-sphere effects, resulting in a smaller R 1,obs . We decided to perform PRE NMR studies on our host-guest complexes to measure binding constants, but instead of measuring the longitudinal relaxation rate of water, we used chloroform as a reporter solvent and acetonitrile as co-solvent to improve guest solubility. Chloroform has been observed in X-ray structures of H 2 1 to reside inside the cavity of the host and thus is an ideal reporter solvent [42] . Acetonitrile was also tested as a reporter solvent, but upon binding it displayed an overall smaller change in the relaxation rate, reducing its reliability. A binding curve was constructed by measuring the relaxation rate of bulk chloroform while varying the guest concentration and keeping the Mn1 concentration constant. 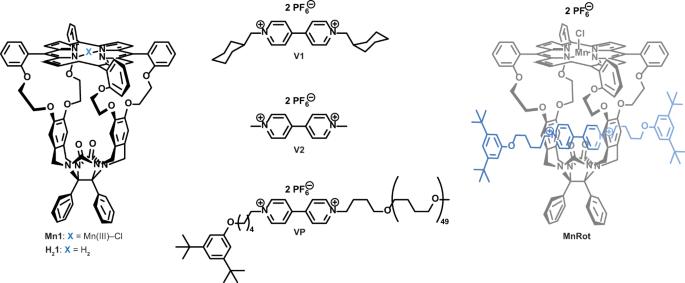Fig. 1: Molecular structures of the studied compounds. Mn(III)-porphyrin cage compoundMn1(porphyrin center atom(s) indicated in blue), bis-(methyl cyclohexyl) viologenV1, methyl viologenV2, polymer-substituted viologenVP, and the rotaxane of a blocked viologen guest (blue) withMn1(MnRot). From these PRE binding titrations, the binding constants of the Mn1 / V1 , Mn1 / V2 , and Mn1 / VP complexes could be determined (Table 1 , for titration curves see Supplementary Fig. 21 ). Table 1 Binding constants of host–guest complexes. Full size table As shown in Table 1 , the log( K a ) of the paramagnetic host–guest complex Mn1 / V1 (3.68 ± 0.16) is significantly lower, i.e., by three orders of magnitude, than that of the diamagnetic host–guest complex H 2 1 / V1 (7.29 ± 0.26). This indicates that H 2 1 / V1 forms a much more stable complex than Mn1 / V1 . This decrease in binding affinity after manganese insertion may be explained by repulsion between the positively charged dicationic viologen guest molecule, and the trivalent metal center which will destabilize the binding of V1 inside the cavity. In this connection it is worth mentioning that the electronic structures of manganese(III) porphyrins, e.g., Mn(III)TPP Cl, have been widely studied in the literature. A partial charge build-up on the metal center was found to occur as a result of the relatively labile Mn−Cl bond [43] , [44] , [45] . As expected, the binding constant for Mn1 / V2 (log( K a ) = 4.20 ± 0.17) was lower than that of the diamagnetic combination H 2 1 / V2 (log( K a ) = 5.78 ± 0.30) [39] . However, V2 binds more strongly inside Mn1 than V1 , whereas the opposite was true for the diamagnetic host H 2 1 . This could be caused by the decrease in sterics when the bulkier methyl cyclohexyl groups on either side of the viologen moiety in V1 are replaced by methyl groups, allowing the resulting guest V2 to be positioned more favorably inside the cavity of Mn1 . This may result in a slight reduction of repulsive interactions between the metal-center and V2 , in contrast to Mn1 / V1 where there is less freedom of movement. Lastly, the binding constant for Mn1 / VP (log( K a ) = 3.23 ± 0.18) was found to be similar in magnitude to Mn1 / V1 (log( K a ) = 3.68 ± 0.16). This is consistent with our previous research where binding constants were determined for H 2 1 and poly-THF substituted viologen guests with variable numbers of monomer units (34–88) [46] , [47] . The obtained binding constants (log( K a ) ~7.4) were very similar to that of the small, symmetric viologen guest V1 with H 2 1 (log( K a ) = 7.29 ± 0.26), indicating that similar (de)stabilizing effects are present. A range of differently metallated porphyrin cages is currently under investigation. A step-by-step how-to guide for determining association constants and dissociation parameters is included in the Supplementary information. Exchange of viologen guests in Mn1 It is evident from Fig. 2 that selective 1 H-NMR experiments, such as 1D EXSY, on host-guest complexes involving Mn1 are not possible due to the excessive broadening of the relevant host resonances. Upon adding ten equivalents of a viologen guest V1 to Mn1 , we can observe a similar paramagnetic-induced broadening of the ortho (8.85 ppm) and meta (8.45 ppm) free guest proton resonances compared to the resonances in the diamagnetic host-free spectrum (Fig. 3a ). Notably, the bound V1 signal is absent, most likely due to a strong R 2 PRE. Fortunately, the limited broadness still allows relaxation experiments to be performed with relative ease on the free guest. Preliminary T 2 measurements revealed a > 16× faster relaxation for V1 (5 mM) in the presence of Mn1 (0.5 mM) compared to the host-free condition (Fig. 3b ). The magnitude of such a large enhancement suggests the occurrence of exchange-based PRE rather than a relaxation enhancement purely caused by the presence of a paramagnetic species in absence of exchange (outer-sphere effects), warranting further investigations [16] . Fig. 3: Influence of the presence of Mn1 on T 2 values of free guest proton signals. a Top: 1 H NMR spectrum of V1 (500 MHz, chloroform- d : acetonitrile- d 3 , 1:1 (v/v), 20 °C), bottom: 1 H NMR spectrum of V1 in the presence of 9 mol% Mn1 (500 MHz, chloroform- d : acetonitrile- d 3 , 1:1 (v/v), 20 °C). b Mono-exponential first order plots of PROJECT-CPMG measurements and the determined T 2 values for the relaxation of the unbound meta-protons of V1 and of V1 in the presence of 9 mol% Mn1 (20 °C), showing an enhancement factor of 16.6×. The color-coding blue and orange refer to the experiments without (diamagnetic) and with (paramagnetic) Mn1 present, respectively. Full size image As described in Eq. 1 , R obs can be divided into a diamagnetic ( R 0 ) and a paramagnetic contribution ( R p ). R p can be further defined as the sum of inner-sphere (close, long-lived binding interactions, \(\frac{{{f}}}{{{{{{{\rm{\tau }}}}}}}_{{{{{{\rm{M}}}}}}}+{{{T}}}_{{{{{{\rm{M}}}}}}}}\) ) and outer-sphere interactions (distant, non-binding interactions, R os ) (see Fig. 4a ). Here, “f” is the the mole-fraction of the ligand bound to the host that takes into account the binding affinity of the guest molecule to the host and the number of binding sites, τ M (s) is the mean-residence time of the guest bound to the host, and T M (s) is the relaxation time constant the guest experiences while bound. By taking the inverse of τ M , the observed dissociation rate constants can be determined and thereby their corresponding energy barriers. When the system falls into a slow-to-intermediate exchange regime with respect to relaxation, τ M can dominate R p under certain conditions and therefore the T M term can be neglected, simplifying the equation to Eq. 2 . R_p=f/τ_M+R_os
 (2) In order to determine if R p is dominated by τ M , and therefore suitable for measuring the rate of dissociation of the guest from the host, three requirements have to be met: 1) R p should increase at higher temperatures ( \(\frac{\partial {{{R}}}_{{{{{{\rm{p}}}}}}}}{\partial {{T}}} \, > \, 0\) ) since τ M would decrease with faster exchange, 2) R p is independent of the field strength ( \(\frac{\partial {{{R}}}_{{{{{{\rm{p}}}}}}}}{\partial {{{{{\rm{\omega }}}}}}}=0\) ) since τ M is field-independent, and 3) R 1,p should approximately be equal to R 2,p ( \(\frac{{{{R}}}_{2,{{{{{\rm{p}}}}}}}}{{{{R}}}_{1,{{{{{\rm{p}}}}}}}}\approx 1\) ) [16] . A more in-depth explanation and justification of the requirements and the simplification of the aforementioned equations can be found in the Supplementary Information. Fig. 4: Determination of relaxation rates of the Mn1/V1 system. a Schematic indication of the different dominating factors governing exchange at different temperatures (low T is left, high T is right). At low temperatures where there is no exchange, the outer-sphere interactions are dominating; at higher temperatures the slow and intermediate exchange regime holds, and the exchange is dominating; and in the fast exchange regime the inner-sphere interactions dominate. The various regimes are indicated in three shades of blue. b Graph of ln( R 1,p ) against the temperature, displaying a positive slope with increasing temperature. The data points for the ortho protons are shown in blue and those for the meta protons in orange. c R 1,p values plotted against temperature comparing 300 MHz (blue dots and blue numbers) and 500 MHz (orange dots and orange numbers) experiments. d Ratio of R 2,p and R 1,p plotted against temperature before (blue dots) and after (orange dots) R 1,os and R 2,os correction. Solvent chloroform- d : acetonitrile- d 3 , 1:1 (v/v). Full size image To determine whether the above requirements are met, the paramagnetic relaxation rates R 1,p and R 2,p of the Mn1 / V1 system were first measured at both 300 and 500 MHz and from 30 to 50 °C. As shown in Fig. 4b–d , all requirements were suitably met within the above temperature range, indicating that τ M was indeed dominating R p . Subsequently, the temperature range was extended to the range −10 to 70 °C in order to be able to assess the kinetics over the largest possible temperature span for an Eyring analysis. When the measurements were performed at lower temperatures, it was observed that the “ \(\frac{{{{R}}}_{2,{{{{{\rm{p}}}}}}}}{{{{R}}}_{1,{{{{{\rm{p}}}}}}}}\approx 1\) ” condition began to deteriorate as R 2,p / R 1,p began to approach 1.5 at −10 °C. This suggested that outer-sphere contributions were playing a larger role in R p as τ M became longer at lower temperatures. To correct for these outer-sphere effects, a manganese rotaxane ( MnRot , Fig. 1 ), where the binding cavity is irreversibly blocked, was synthesized (see Supplementary Information), and R 1,obs and R 2,obs were measured under identical conditions for MnRot/V1 over the complete temperature range. After correcting for the outer-sphere interactions, the “ R 1,p ≈ R 2,p ” condition proved to be satisfactory held over the complete temperature range (Fig. 4d ). By measuring R obs , R 0 , and R os the observed dissociation rate constant ( k d,obs ) for V1 could be calculated using Eqs. 1 and 2 (Tables S8 and S9 ). To calculate the actual dissociation rate constant ( k d ), the observed dissociation rate constant has to be corrected for the host and guest dependence on the residence time of the ligand near or on the metal ( τ M ). If both the host and guest concentration have no influence on τ M , k d,obs will be equal to k d . However, if there is an additional host or guest dependence on the residence time, the k d,obs will have to be corrected for the order of the dependence. We determined the host and guest dependence on the exchange by measuring the residence time of the guest in the V1 / Mn1 complex at different V1 and Mn1 concentrations (see Supplementary Table 7 ). From these experiments an exchange-promoting behavior was found when the guest concentration was increased. However, the exchange process was characterized by a non-integer order (~0.3). When the measurements were repeated for Mn1 and a guest similar to V1 (Supplementary Fig. 2b ), again a non-integer order (~0.4) was obtained. To determine whether this guest dependence resulted from a guest or a host effect, EXSY experiments were performed on the diamagnetic H 2 1 / V1 complex (Supplementary Figs. 23 and 24 ) [36] . In this case, a zero-order guest dependence was found (Supplementary Fig. 2c ), indicating that the presence of the manganese metal inside the porphyrin ring significantly alters the mechanism for guest dissociation. The observed non-integer dependence can have different origins: the possible additional binding of a guest molecule on the outside of the porphyrin cage could promote dissociation, the counter ions of the viologen salt (hexafluorophosphates) could play a role by exchanging with Cl − ions, which may influence the ability for the guest to dissociate, and, finally, a combination of associative and dissociative mechanisms may occur. These mechanistic explanations are interesting and require further studies, which are underway. Our primary interest, however, was the determination of the activation parameters for guest dissociation from the host–guest complex. 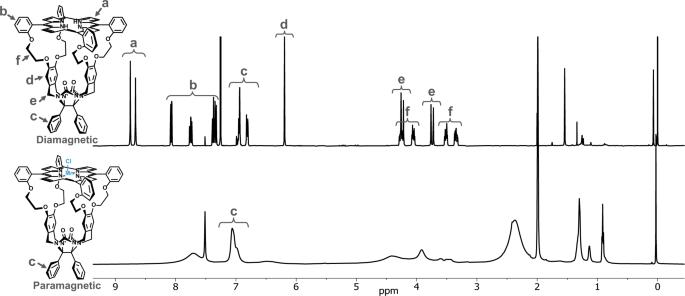Fig. 2: Influence of the presence of a paramagnetic Mn center on the1H NMR spectrum of a host compound. Top:1H NMR spectrum of metal-free porphyrin cage compoundH21(500 MHz, chloroform-d: acetonitrile-d3, 1:1 (v/v), 25 °C), bottom:1H NMR spectrum ofMn1(500 MHz, chloroform-d: acetonitrile-d3, 1:1 (v/v), 25 °C) (metal center and counter ion in blue). After correcting k d,obs for the guest dependence, the activation energies (Δ H ‡ , Δ S ‡ , and Δ G ‡ ) were extracted from the Eyring plots (Table 2 and Supplementary Fig. 20 ). Table 2 Activation enthalpies, entropies and free energies of dissociation for different host–guest complexes. Full size table In order to assess the influence of Mn(III) Cl insertion into the porphyrin ring we may compare the activation energy barriers for dissociation of the Mn1 / V1 system with those of the diamagnetic system H 2 1 / V1 . Interestingly, the Δ G ‡ of the Mn1 / V1 complex is substantially lower (13.59 ± 0.17 kcal mol −1 ) than that of the diamagnetic host–guest complex H 2 1 / V1 (17.99 ± 0.43 kcal mol −1 ). The difference of ~4.5 kcal mol −1 in ΔΔ G ‡ mirrors the ~5 kcal mol −1 difference in ΔΔ G (Table 1 ), suggesting that ground-state effects play a significant role in lowering the activation energies for exchange when a Mn(III) ion is inserted into the porphyrin of the cage compound. The PRE experiments were repeated with Mn1 and viologen polymer VP . This guest molecule has been studied previously with H 2 1 , where it was confirmed that threading and exchange do occur [36] . We previously had expected and assumed that polymers would thread through Mn1 [47] , [48] , but PRE NMR studies now offer the possibility to definitively prove whether this hypothesis holds true. For the Mn1 / VP system R obs should be compared to R os . Here, R obs is measured by a sample containing Mn1 and VP , and for R os a sample containing MnRot and VP . If R obs ≈ R os then the inner-sphere contribution is near-zero and there will be (almost) no exchange and, consequently, possibly no threading. If the observed relaxation rate is much larger than the outer-sphere contribution ( R obs ≫ R os ), then this supports that exchange and hence threading occurs. We performed these PRE NMR experiments and found that the observed relaxation rates ( R 1,obs = 11.94 s −1 , R 2,obs = 10.02 s −1 ) indeed are significantly larger than the outer-sphere contributions ( R 1,os = 1.03 s −1 , R 2,os = 1.38 s −1 ), i.e., by approximately a factor of nine, which is in a similar order of magnitude as found for Mn1 / V1 . These experiments, therefore, demonstrate that Mn1 indeed threads VP . From the Eyring plot (Fig. S20c, d ) the activation energy barriers for dissociation could be determined (Table 2 ), and similar energy barriers were observed for Mn1 / VP (13.92 ± 0.40 kcal mol −1 ) compared to Mn1 / V1 (13.59 ± 0.17 kcal mol −1 ). The notion that the destabilized binding of V1 in the cavity of Mn1 results in facile dissociation and therefore faster exchange is further confirmed by the measured binding constants of Mn1 / VP ( K a = 1692 ± 295 M −1 ) and Mn1 / V1 ( K a = 4796 ± 769 M −1 ), which are in the same order of magnitude. Furthermore, since chloroform exposure to the cavity was the observable feature in the binding studies, these experiments directly point to complete dissociation of the polymer as opposed to a slipping process in which the viologen moiety slips in and out of the cavity without full dissociation of the polymer-chain. From the measured energy barriers for exchange (Δ H ‡ = 3.17 ± 0.33 kcal mol −1 , Δ S ‡ = −36.89 ± 3.29 cal K −1 mol −1 ) it is evident that for the Mn1/VP system the dissociation is almost entirely governed by entropy. Possible reasons for the high entropy contribution to the dissociation of the polymer could be linked to the notion that a significant extent of order should be achieved for complete dissociation of a molecule with this length. It could also be influenced by the resolvation of the polymer chain after dissociation or possible wrapping of the polymer-chain around the porphyrin host [37] . The significantly lower activation enthalpy (Δ H ‡ = 3.17 ± 0.33 kcal mol −1 ) found for Mn1 / VP compared to Mn1 / V1 (Δ H ‡ = 8.35 ± 0.17 kcal mol −1 ) may be attributed to the possibility that the viologen-moiety of VP is threaded, but not deeply bound inside the cavity of Mn1 , as opposed to Mn1 / V1 , resulting in a lower dissociation activation enthalpy for Mn1 / VP . Another possibility is the difference in sterics between V1 and VP . The observed higher Δ H ‡ of the former compound may be a result of the presence of the bulkier methyl cyclohexyl substituents on either side of its viologen moiety compared to the unbranched carbon chains attached to that of VP , possibly complicating dissociation. To test the latter theory and to see if the activation enthalpy would be lower, the PRE NMR measurements were repeated with methyl viologen V2 (see Supplementary Information p 35–40). Here, similar Δ H ‡ values for the dissociation of Mn1 / V2 (7.99 ± 1.08 kcal mol −1 ) compared to that of Mn1 / V1 (8.35 ± 0.17 kcal mol −1 ) were found, rejecting the hypothesis that less bulky substituents on the viologen guest result in lower activation enthalpies. Hence, we attribute the appreciable difference in dissociation Δ H ‡ values measured for Mn1 / V1 and Mn1 / VP to an increase in statistical host positions on the polymer chain, as opposed to Mn1 / V1 where the viologen moiety is deeply bound inside the cavity of its host. Lastly, from the now known k d values of Mn1 / VP (Supplementary Tables 10 and 11 ) and the previously determined binding constant, threading rate constants ( k on ) can be calculated from \({{{K}}}_{{{{{{\rm{a}}}}}}}=\frac{{{{k}}}_{{{{{{\rm{on}}}}}}}}{{{{k}}}_{{{{{{\rm{d}}}}}}}}\) and be used to construct an Eyring plot from 20 to 70 °C, from which activation energies can be extracted. Here, it is assumed that the binding constant of Mn1 / VP remains relatively insensitive to the temperature (see Supplementary Fig. 22 ). 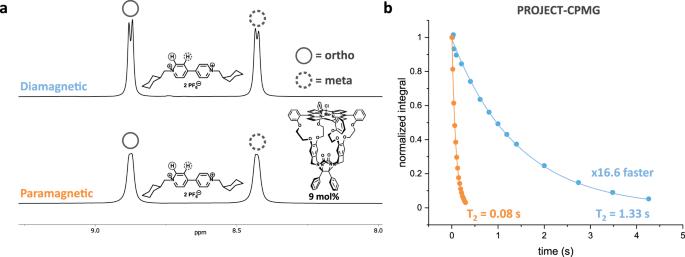Fig. 3: Influence of the presence of Mn1 onT2values of free guest proton signals. aTop:1H NMR spectrum ofV1(500 MHz, chloroform-d: acetonitrile-d3, 1:1 (v/v), 20 °C), bottom:1H NMR spectrum ofV1in the presence of 9 mol%Mn1(500 MHz, chloroform-d: acetonitrile-d3, 1:1 (v/v), 20 °C).bMono-exponential first order plots of PROJECT-CPMG measurements and the determinedT2values for the relaxation of the unbound meta-protons ofV1and ofV1in the presence of 9 mol%Mn1(20 °C), showing an enhancement factor of 16.6×. The color-coding blue and orange refer to the experiments without (diamagnetic) and with (paramagnetic)Mn1present, respectively. 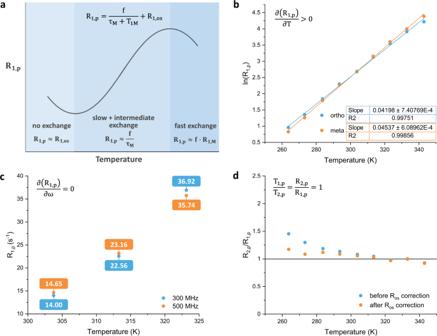Fig. 4: Determination of relaxation rates of the Mn1/V1 system. aSchematic indication of the different dominating factors governing exchange at different temperatures (lowTis left, highTis right). At low temperatures where there is no exchange, the outer-sphere interactions are dominating; at higher temperatures the slow and intermediate exchange regime holds, and the exchange is dominating; and in the fast exchange regime the inner-sphere interactions dominate. The various regimes are indicated in three shades of blue.bGraph of ln(R1,p) against the temperature, displaying a positive slope with increasing temperature. The data points for the ortho protons are shown in blue and those for the meta protons in orange.cR1,pvalues plotted against temperature comparing 300 MHz (blue dots and blue numbers) and 500 MHz (orange dots and orange numbers) experiments.dRatio ofR2,pandR1,pplotted against temperature before (blue dots) and after (orange dots)R1,osandR2,oscorrection. Solvent chloroform-d: acetonitrile-d3, 1:1 (v/v). The calculated threading parameters for Mn1 / VP are listed in Table 3 , together with threading parameters from previous studies in which the threading of H 2 1 onto variable-length poly-THF substituted viologens was studied. It is apparent from Table 3 that Mn1 / VP surprisingly threads faster ( k on = (4.66 ± 1.04) × 10 5 M −1 s −1 ) than combinations of VP with the metal-free host ( k on = (1.9–3.6) × 10 4 M −1 s −1 ) [46] . Analysis of the Eyring parameters reveals that the difference between the threading of VP through Mn1 and through H 2 1 is solely enthalpic in nature, as the entropy values are very similar. We tentatively ascribe this to a pre-binding effect, which has been proposed in earlier work [47] , [49] . It involves a preassociation of the porphyrin cage with the polymer and diffusion along its chain, allowing the polymer end to loop back into the cavity of the host (effective molarity effect), aiding the threading process. We suggest that this process is more effective for Mn1 / VP than for H 2 1 / VP because of the positive charge residing on the Mn1 center, interacting stronger with the oxygen atoms in the polymer chain. Furthermore, the interaction of the polymer end with the cavity of the cage, which initiates the threading process (entron effect) [47] , will be stronger for Mn1 than for H 2 1 . The above mechanism explains why the Δ S ‡ values for Mn1 / VP and H 2 1 / VP are similar, but the Δ H ‡ value is lower for Mn1 . Table 3 k on values and threading parameters for Mn1/VP, and reference parameters for H 2 1 with comparable poly-THF substituted viologen guests. Full size table We have shown that paramagnetic relaxation enhancement experiments can be utilized to investigate chemical exchange binding strength in the field of metallohost–guest chemistry for systems displaying both slow to medium exchange rates (utilized to measure dissociation) and fast exchange rates (utilized to perform association titrations), even if the resonances corresponding to the bound species are not directly visible. Binding titration studies revealed that a paramagnetic host–guest complex, involving a manganese(III) metal in the porphyrin ring of the cage compound, displays significantly lower binding affinities for viologen guests compared to those of the non-metallated porphyrin cage with the same guest compounds. Furthermore, Mn1/V1 displays lower energy barriers for guest dissociation compared to H 2 1 / V1 . The combined results of lower binding constants and lower dissociation barriers for Mn1 / V1 compared to H 2 1 / V1 indicate that for the paramagnetic system ground-state effects play an important factor in the decrease of the activation barriers for dissociation. These destabilizing effects may be caused by repulsive interactions between the positively charged metal center and the dicationic viologen guest. Furthermore, decreasing the bulkiness on the substituents of the guest compound (compare Mn1 / V2 versus Mn1/V1 ) resulted in slightly stronger binding and faster dissociation, which likely is a result of the increased freedom of movement of the guest inside the cavity of the host in combination with decreased steric interactions. The PRE studies could also be performed on the host–guest complex Mn1 / VP , which involves a polymer chain to which a viologen moiety is attached. The much larger value observed for the relaxation rates ( R 1,obs = 11.94 s −1 , R 2,obs = 10.02 s −1 ) compared to the outer-sphere contributions ( R 1,os = 1.03 s −1 , R 2,os = 1.38 s −1 ) presents irrefutable evidence that Mn1 is capable of threading VP , confirming a long-standing hypothesis. Surprisingly, the threading rate of Mn1 onto VP was found to be considerably faster than that of the non-metallated porphyrin cage H 2 1 onto VP . We attribute this to a pre-association of the positively charged Mn1 complex to the outside of the oxygen-containing poly-THF chain, allowing the polymer end to loop back and find the cavity of Mn1 more easily (effective molarity effect). The methodology presented in this paper provides a blueprint for how binding and dynamics in other paramagnetic systems, especially catalytic ones, which are extensively studied in the field of organic chemistry, could be thoroughly investigated. Longitudinal relaxation rates were measured through inverse recovery experiments and transverse relaxation rates were measured via by utilizing the CPMG [50] , [51] (Carr-Purcell-Meiboom-Gill) pulse sequence and the PROJECT-CPMG [52] (Periodic Refocusing of J Evolution by Coherence Transfer CPMG) sequence on a Bruker 500 MHz Avance III spectrometer equipped with a Prodigy BB cryoprobe or a Bruker 300 MHz Avance III HD nanobay spectrometer equipped with a BBFO probe. For all VT experiments, the temperature was calibrated using pure ethylene glycol for temperatures of 20 °C and higher. Methanol was used to calibrate the temperatures lower than 20 °C. Fluorescence quenching titrations were performed on a JASCO FP-8300ST Spectrofluorometer in a quartz cuvette with 1 cm path length. Samples for titrations consisted of anhydrous chloroform and anhydrous acetonitrile (1:1, v/v). Anhydrous chloroform (>99%) and acetonitrile were obtained from Sigma-Aldrich. Before use, the chloroform was filtered over dry K 2 CO 3 and acetonitrile was distilled and dried over CaCl 2 . For all titration studies, which were carried out at 22 °C, the solutions were irradiated with light of 419 nm.